Overcoming ultraviolet light instability of sensitized TiO2with meso-superstructured organometal tri-halide perovskite solar cells The power conversion efficiency of hybrid solid-state solar cells has more than doubled from 7 to 15% over the past year. This is largely as a result of the incorporation of organometallic trihalide perovskite absorbers into these devices. But, as promising as this development is, long-term operational stability is just as important as initial conversion efficiency when it comes to the development of practical solid-state solar cells. Here we identify a critical instability in mesoporous TiO 2 -sensitized solar cells arising from light-induced desorption of surface-adsorbed oxygen. We show that this instability does not arise in mesoporous TiO 2 -free mesosuperstructured solar cells. Moreover, our TiO 2 -free cells deliver stable photocurrent for over 1,000 h continuous exposure and operation under full spectrum simulated sunlight. Titanium dioxide (TiO 2 ) nanoparticles have long been considered promising materials for energy storage, photocatalysis and photovoltaic technologies [1] , [2] , [3] , [4] . Sensitized solar cells (SSCs), where mesoporous TiO 2 is used as the electron transporter, have reached close to commercial power conversion efficiencies of 12.3% using a liquid electrolyte and porphyrin dyes [5] , and up to 15% with solid-state hole transporters and organometal halide perovskite absorbers [6] , [7] , [8] , [9] . In addition, organometal halide perovskites are capable of transporting both electrons and holes [8] , [10] , and operate efficiently in a planar p–i–n heterojunction configuration [11] , delivering over 15% efficiency [12] . When CH 3 NH 3 PbI 3− x Cl x is coated onto an insulating alumina scaffold, it can yield performances of up to 12.3% in a mesoporous TiO 2 -free hybrid solar cell, which we term a meso-superstructured solar cell (MSSC) [8] , [11] . These solid-state approaches have the advantage that they do not suffer from electrolyte leakage, nor does the hole-transporting material (HTM) possess any corrosive qualities that we know of [1] , [13] , [14] . As the efficiency is likely to increase and become comparable with the best thin-film and wafer-based technologies, a critical challenge for global adoption of perovskite-based solar cells is the proof or realization of longevity. Realizing stable modules is an industrial task, largely down to effective encapsulation and module design, rather than a fundamental academic task. However, ensuring that the basic chemistry from which the technology is constructed is fundamentally stable will reduce the subsequent industrial effort required and greatly help the technology enter the market. Considering the importance of a solar cell’s long-term stability and the premise of solid-state SSCs delivering superior stability than the liquid electrolyte counterparts, there is very little published research on the topic [6] , [15] , [16] , [17] , [18] . The studies which have been conducted to date for solid-state dye-sensitized and perovskite-SSCs are not clear in the exact nature of encapsulation, nor on the precise ageing and testing conditions [6] , [8] , [9] , [15] , [16] , [18] . In addition, ultraviolet (UV) cutoff filters are often used, but the effect of UV light on solar cell stability is not yet well understood [6] , [8] , [9] , [15] , [16] , [18] . In contrast, a great deal of literature is available on the subject of long-term stability of polymer-based solar cells, which require encapsulation to protect the organic components from oxidation in air [19] , [20] , [21] , [22] . Air sensitivity of organics, coupled with the moisture sensitivity of the current generation of perovskite absorbers, makes it clear that this new class of solar cells will require a high level of encapsulation to attain eventual outdoor lifetimes of over 25 years [6] , [8] , [23] . A number of previous reports on solid-state dye-sensitized solar cells (DSSCs) elude to significant performance deteriorations when operated in an inert atmosphere. This has been assigned to changes in the metal oxide surface and changes to the level of p-doping in the hole transporter [17] , [24] , [25] , [26] . With this in mind, we have performed a series of aging tests on TiO 2 -SSCs using both dye-sensitizers (an indolene dye termed D102 and a ruthenium complex dye termed C106) and the methylammonium lead iodide chloride mixed halide perovskite absorber CH 3 NH 3 PbI 3− x Cl x in different environments. The TiO 2 -SSCs encapsulated in a nitrogen atmosphere suffer from an extremely rapid (30 min half-life) decay in photocurrent and performance under simulated sunlight with the full UV component present. We describe the mechanism driving this drop in performance and propose that oxygen serves to pacify deep electronic trap sites at oxygen vacancies in the TiO 2 . The simplest and surest means to remove the deep trap sites is to entirely remove the mesoporous TiO 2. Indeed we demonstrate that the high efficiency MSSCs exhibit extremely stable photocurrent over 1,000 h of continuous full spectrum AM1.5 solar illumination at 40 °C (<10% change after a slight rise in the first 10 h). This identifies a key advantage of the MSSC; not only does it deliver fundamentally higher efficiency, but removal of the mesoporous TiO 2 also sidesteps a critical instability. UV light induced degradation of TiO 2 -based solar cells To investigate the UV aging effect on the perovskite-based solar cells, we have exposed a variety of different solar cell configurations to 5 h of simulated AM 1.5 100 mW cm −2 sunlight without any additional UV filtration. 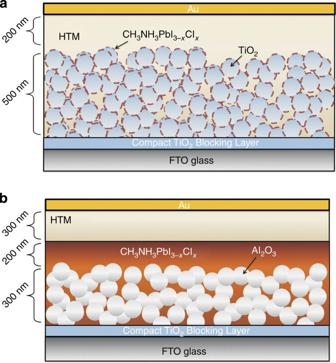Figure 1: Solar cell architectures. (a) Depiction of a solar cell made by sensitizing mesoporous TiO2with the mixed halide perovskite absorber. This active layer is then infiltrated with spiro-OMeTAD as HTM. (b) Schematic of a solar cell where the perovskite itself is functioning as both light absorber and electron transporter. The Al2O3is functioning as a scaffold to enhance film formation, while the spiro-OMeTAD HTM is functioning as a hole extraction layer. Figure 1 depicts the solar cell structures used. Figure 1a shows a cell composed of a 500-nm mesoporous TiO 2 active layer sensitized by the perovskite absorber and infiltrated with the 2,2′ 7,7′-tetrakis-(N,N-di-p-methoxyphenylamine)-9,9′-spirobifluorene (spiro-OMeTAD) HTM, while Fig. 1b shows the structure of our current most efficient MSSC, where a thin inert alumina scaffold is used to allow the formation of a thin solid perovskite-capping layer which forms a planar heterojunction with the spiro-OMeTAD HTM. The first structure, where the perovskite is acting as a sensitizer (we verify that the CH 3 NH 3 PbI 3− x Cl x is present only as a thin layer on the TiO 2 nanoparticles in Supplementary Fig. S1 and Supplementary Note 1 ), relies on electron transport through TiO 2 (refs 6 , 8 ), while the second structure functions more similarly to a thin film p-i-n heterojunction solar cell where charge is generated and electrons and holes are transported within the perovskite layer [8] , [11] , [12] . We point out that we use gold electrodes here rather than silver, because we have previously demonstrated that silver contacts often form shunting paths with the mesoporous TiO 2 in the absence of oxygen [17] . In addition, the silver can become corroded when in contact with the perovskite film, which is likely to be due to the formation of silver halide. Figure 1: Solar cell architectures. ( a ) Depiction of a solar cell made by sensitizing mesoporous TiO 2 with the mixed halide perovskite absorber. This active layer is then infiltrated with spiro-OMeTAD as HTM. ( b ) Schematic of a solar cell where the perovskite itself is functioning as both light absorber and electron transporter. The Al 2 O 3 is functioning as a scaffold to enhance film formation, while the spiro-OMeTAD HTM is functioning as a hole extraction layer. Full size image In Fig. 2 , we show the evolution of solar cell performance parameters over time under illumination for TiO 2 -based perovskite-SSCs, measured in air, encapsulated in a nitrogen-filled glove box, and encapsulated but with the additional filtration of the UV component of the light by using a 435-nm UV cutoff filter. Initial performance parameters of the devices are given in Supplementary Table 1 . Surprisingly, the encapsulated sensitized TiO 2 cells decay much faster than the non-encapsulated solar cells when subjected to full spectrum sunlight, falling to less than 10% of their initial performance within 5 h due to a rapid decrease in photocurrent and a smaller decrease in photovoltage. This is in contrast to only 50% decay over 5 h illumination for the non-encapsulated devices tested in ambient conditions. When a UV filter (435 nm cutoff) is used, however, the solar cells are more stable, with the encapsulated sensitized TiO 2 cells decaying to only 85% of their initial performance within the 5 h. Notably for the UV-filtered devices (435 nm cutoff), the degradation of the photocurrent is diminished (but still present), while the photovoltage stays constant and the fill factor decreases slightly. The fill factor drop may simply be due to non-optimum doping of the HTM [15] . We note that we also observe a similar rapid drop in photocurrent in solid-state DSSCs using either a ruthenium complex dye or an organic dye upon encapsulation in an inert atmosphere and exposure to a significant component of UV illumination ( Supplementary Figs S2 and S3 , Supplementary Note 2 ). This suggests that the problem does not lie with the perovskite absorber material, but elsewhere. The fact that there is no change in the UV–vis spectra of the solar cells over this time period is further evidence ( Supplementary Fig. S4 ) that the absorber material is not degrading. We note that there has also been interest in using the organolead trihalide perovskites to fill the pores of the TiO 2 simply by increasing the precursor solution concentration ( Supplementary Fig. S5 ), so that it acts as both a sensitizer and a hole transporter [7] , [10] , [23] . We find that this structure is also unstable upon encapsulation when exposed to unfiltered simulated sunlight, though with a slower decay, decaying to 50% of the initial performance over the course of 5 h full spectrum illumination ( Supplementary Fig. S5 and Supplementary Note 3 ). 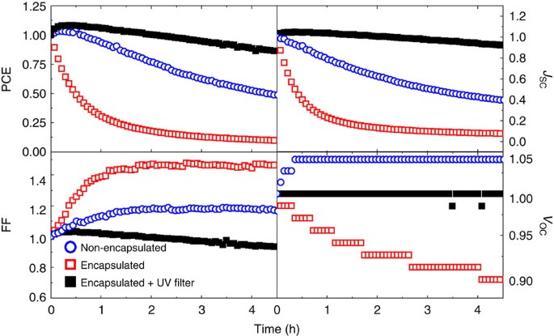Figure 2: Aging of TiO2-based solar cells. Evolution of normalized solar cell performance parameters, power conversion efficiency , short circuit current (Jsc), fill factor (FF), and open circuit voltage (Voc) over 5 h of AM1.5 100 mW cm−2solar illumination. We compare the behaviour of perovskite-sensitized TiO2solar cells which are non-encapsulated (blue open circles) and encapsulated with (filled black squares) and without a<435-nm cutoff filter (open red squares). We note that all devices had initial power conversion efficiencies of at least 5%, with short circuit currents of at least 10 mA cm−2, representing typical working solar cells of this type. Figure 2: Aging of TiO 2 -based solar cells. Evolution of normalized solar cell performance parameters, power conversion efficiency , short circuit current ( J sc ), fill factor (FF), and open circuit voltage ( V oc ) over 5 h of AM1.5 100 mW cm −2 solar illumination. We compare the behaviour of perovskite-sensitized TiO 2 solar cells which are non-encapsulated (blue open circles) and encapsulated with (filled black squares) and without a<435-nm cutoff filter (open red squares). We note that all devices had initial power conversion efficiencies of at least 5%, with short circuit currents of at least 10 mA cm −2 , representing typical working solar cells of this type. Full size image Others have ascribed the poor performance of solid-state DSSCs in the absence of oxygen to insufficient p-doping of the spiro-OMeTAD hole transporter [24] , [25] , [27] . However, we have previously demonstrated that once the oxidation reaction is complete, the p-doping of the hole transporter is predominantly stable even when placed in an oxygen free atmosphere [25] . So we do not expect that de-doping of the hole conductor is primarily responsible for the performance drop upon encapsulation. We demonstrate the implications of this on preparing and testing solid-state DSSCs in an oxygen free environment in detail in Supplementary Fig. S6 and Supplementary Note 4 ). Evidence for deep electron trapping in aged TiO 2 -based solar cells In an attempt to determine whether the drop in photocurrent is caused by deterioration in charge generation or charge collection, we have performed simultaneous charge extraction (at short circuit) and transient absorption spectroscopy (TAS) on complete solar cells with semi-transparent electrodes (15 nm gold), using a 550-nm laser pulse as the excitation. We have previously used this method to quantify the extinction coefficient of oxidized spiro-OMeTAD in devices we know to have near unity charge collection efficiency [27] . Here, we use this technique to simultaneously monitor the decay of the oxidized spiro-OMeTAD signal and the decay of the photocurrent following a light pulse, before and after degradation of the sealed TiO 2 -based solar cells. From this, we can determine the ratio of charges generated (G, determined from the early time oxidized spiro-OMeTAD absorption signal) to the total number of charges collected (C, determined from the time integrated short-circuit photocurrent perturbation). The ratio between the charges generated (G) to those collected (C) is a direct measurement of the collection efficiency (C/G × 100%). In Fig. 3a we show the transient short-circuit photocurrent trace, and in Fig. 3b we show the transient absorption signal. The table inset to Fig. 3a gives the calculated values for G, C and charge collection efficiency. For this analysis, we assume that the number of holes in spiro-OMeTAD is equivalent to the number of electrons in the TiO 2 , which we will verify later. 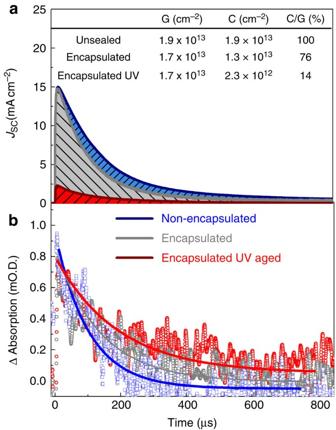Figure 3: Current extraction and transient absorption spectroscopy of TiO2-based solar cells. In the top panel (a), the current collected from full perovskite-sensitized TiO2solar cells with semitransparent electrodes (15 nm gold) after a 10 ns laser pulse (550 nm) is plotted against time after the excitation. Non-encapsulated (blue), encapsulated after ambient light exposure (grey) and encapsulated after UV aging (red) (5 min at 40 mW cm−2, 365 nm) are compared. The area underneath the curves represent the total amount of collected charge. In the bottom panel (b), the transient absorption trace at short circuit of the hole on spiro-OMeTAD is probed at 510 nm, performed simultaneously with the current extraction. The lines are merely guides to the eye. The table inFigure 3shows the charge generated (G, estimated from the early time transient absorption sigmal), collected (C, by integrating the current decay), and the ratio between the two as a percentage (C/G). The laser intensity was 80 μJ cm−2, giving charge densities similar to those found in devices under operating conditions27. Figure 3: Current extraction and transient absorption spectroscopy of TiO 2 -based solar cells. In the top panel ( a ), the current collected from full perovskite-sensitized TiO 2 solar cells with semitransparent electrodes (15 nm gold) after a 10 ns laser pulse (550 nm) is plotted against time after the excitation. Non-encapsulated (blue), encapsulated after ambient light exposure (grey) and encapsulated after UV aging (red) (5 min at 40 mW cm −2 , 365 nm) are compared. The area underneath the curves represent the total amount of collected charge. In the bottom panel ( b ), the transient absorption trace at short circuit of the hole on spiro-OMeTAD is probed at 510 nm, performed simultaneously with the current extraction. The lines are merely guides to the eye. The table in Figure 3 shows the charge generated (G, estimated from the early time transient absorption sigmal), collected (C, by integrating the current decay), and the ratio between the two as a percentage (C/G). The laser intensity was 80 μJ cm −2 , giving charge densities similar to those found in devices under operating conditions [27] . Full size image The charge collection efficiency for the unsealed device is approximately unity. Upon sealing and subsequent measuring, there is a moderate decrease in the estimated charge collection efficiency to 76%, but continuous exposure to the 550-nm laser for an hour does not result in further deterioration. In contrast, subsequent exposure of the same cells (encapsulated UV aged) to 5 min of 365-nm light (40 mW cm −2 ) results in a substantial drop of the photocurrent extraction by close to a factor of 7 with the collection efficiency dropping to 14%. By simultaneously monitoring the absorption of oxidized spiro-OMeTAD ( Fig. 3b ) while these photocurrent extraction measurements are performed, we observe that the number of generated charges are not strongly affected by the encapsulation or the UV exposure. In addition, the decay lifetime of the oxidized spiro-OMeTAD signal at short circuit is also not sped up, but actually somewhat slowed down. Since the short circuit TAS decay is a superposition of charge collection and recombination, we cannot readily infer detailed information from this change in rate of decay. To understand the nature of the decrease in collection efficiency and gain an insight into electronic changes in the photoactive layer, we have performed small perturbation photocurrent and photovoltage decay measurements before and after UV light exposure ( Supplementary Fig. S7 and Supplementary Note 5 ) [28] . We find that at a given background light intensity, there is no discernible change in the charge transport lifetime, whereas recombination lifetimes appear to become slightly (factor of 2) longer after UV aging. This is at odds with the direct measurement of the collection efficiency presented in Fig. 3 , since the transient measurements would suggest an increase in the charge collection efficiency. To account for the lost charge after UV aging, we propose that the UV-degraded cells suffer from a deep trapping of injected electrons within newly available sites in the TiO 2 . The photocurrent extraction measurements suggest that these trapped electrons are immobile, while the TAS ( Fig. 3b ) shows that they recombine with oxidized spiro-OMeTAD species on the μs–ms time-scale. The charge that is collected must still be transported via the accepted trap-limited diffusion process through shallow trap sites in the TiO 2 , distinct from the deep UV generated traps, explaining the negligible change in transport lifetimes and hence electron diffusion lengths determined via small perturbation photocurrent decay measurements. If a large portion of the injected electrons in the TiO 2 are indeed deeply trapped and immobile, as we have suggested, then we should be able to confirm this via time resolved conductivity measurements. We have recently introduced a new technique, where we combine conductivity measurements of dye-sensitized TiO 2 with TAS [27] . We now use this technique to observe the effects of UV aging on the conductivity of electrons injected into the TiO 2 by a sensitizer. Using a sensitizing dye (C106), rather than the perovskite sensitizer, allows us to monitor the photobleach of the ground state absorption of the dye to gain a quantitative insight into the density of injected electrons. This is a valid substitution, since the encapsulated solid-state DSSCs degrade similarly to the perovskite-sensitized cells under illumination ( Supplementary Fig. S2 ). The absence of a hole transporter or the perovskite allows us to be confident that we are measuring electron conductivity in the TiO 2 only. 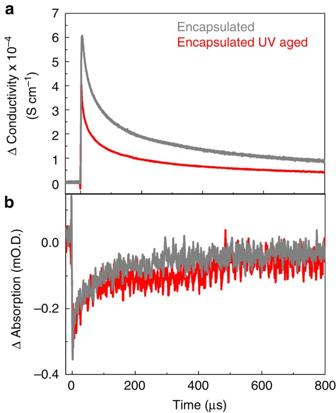Figure 4: Photoinduced change in conductivity and transient absorption of dye-sensitized TiO2. (a) The photoinduced change in conductivity of dye-sensitized TiO2, measured after a 10 ns laser excitation (550 nm at 80 μJ cm−2), and (b) simultaneous transient absorption spectroscopy to monitor the bleach of the dye ground state absorption at 500 nm. Grey corresponds to the encapsulated sample before UV exposure, while the red trace corresponds to the same sample after 5 min UV exposure (40 mW cm−2at 365 nm). Figure 4 shows the laser pulse induced increase in conductivity ( Fig. 4a ), and the transient absorption traces monitoring the bleach at the dye absorption peak of 500 nm ( Fig. 4b ) before and after UV exposure of encapsulated TiO 2 conductivity samples. The first noticeable difference before and after UV light exposure is the increase in absolute background conductivity ( t <0) after aging ( Supplementary Fig. S8 and Supplementary Note 6 ). One would expect such an increase in background conductivity to represent a filling of the TiO 2 sub-bandgap states, increasing the electron mobility [27] , [29] , [30] , [31] . The UV aging in absence of oxygen should then result in an increased mobility and overall conductivity for injected electrons. However, from Fig. 4a,b it is apparent that although the number of electrons injected into the TiO 2 upon excitation of the dye does not change, the resulting photoinduced increase in conductivity is significantly less for the UV-aged samples. We propose that this is because a large fraction of injected electrons are deeply trapped (either directly or after injection on a time scale much faster than our resolution in the TAS (<10 ns)) and do not contribute to the measured conductivity. We have performed the same experiment, but infiltrating the dye-sensitized TiO 2 with spiro-OMeTAD as hole conductor to monitor the photoinduced conductivity change in spiro-OMeTAD. The data is presented in the Supplementary Information , and demonstrate negligible change in the photoinduced conductivity of the hole transporter after UV aging, while the recombination rate is increased ( Supplementary Fig. S9 and Supplementary Note 7 ). The combined measurements on dye-sensitized TiO 2 with and without the hole transporter give a clear picture of what is occurring: photoinduced electron transfer to TiO 2 and hole transfer to spiro-OMeTAD are largely unaffected, but a large fraction of the electrons injected into TiO 2 are trapped in deep trap sites and are not collected but eventually recombine with holes in the spiro-OMeTAD, consistent with our previous hypothesis. Figure 4: Photoinduced change in conductivity and transient absorption of dye-sensitized TiO 2 . ( a ) The photoinduced change in conductivity of dye-sensitized TiO 2 , measured after a 10 ns laser excitation (550 nm at 80 μJ cm −2 ), and ( b ) simultaneous transient absorption spectroscopy to monitor the bleach of the dye ground state absorption at 500 nm. Grey corresponds to the encapsulated sample before UV exposure, while the red trace corresponds to the same sample after 5 min UV exposure (40 mW cm −2 at 365 nm). Full size image To justify the degradation mechanism, we consider the surface chemistry of TiO 2 . TiO 2 is known to contain many oxygen vacancies (or Ti 3+ sites), particularly at the surface, which are effectively deep electron-donating sites [32] , [33] . The electrons in these sites, at approximately 1 eV below the conduction band edge [34] , interact with molecular oxygen in the atmosphere, which adsorbs to the oxygen vacancy sites [35] , [36] , [37] , [38] . As a result, a charge transfer complex (O 2 − –Ti 4+ ) is formed [37] , [38] , [39] , [40] . On the basis of previous work on oxygen adsorption on TiO 2 surfaces [32] , [33] , [35] , [36] , [37] , [38] , [39] , [40] and on our findings here, we propose that the mechanism illustrated in Fig. 5 is responsible for the photocurrent degradation in the solar cells. Upon bandgap excitation of TiO 2 , an electron-hole pair is formed. The hole in the valence band has been shown to recombine with the electron at the oxygen adsorption site, desorbing the oxygen [39] , [40] . This leaves a free electron in the conduction band and a positively charged, unfilled oxygen vacancy site at the TiO 2 surface. Since spiro-OMeTAD is heavily p-doped when used as the HTM in such solar cells, there are excess holes (more than the photogenerated hole density at one sun), which will readily recombine with the free electron left behind from the bandgap excitation of the TiO 2 (refs 24 , 25 , 27 ). We propose that it is in the now unfilled deep trap sites that the lost photoinduced electrons are trapped, and from which they recombine with holes in spiro-OMeTAD [41] , [42] , [43] . Since the rate of oxygen desorption (and hence activation of these trap sites) is likely to be low and reversible [39] , [40] , the steady-state number of empty deep trap sites will be dependent upon the partial pressure of oxygen in the pores, and hence far lower in the presence of oxygen than in the absence of oxygen. By this means, oxygen serves to pacify these sites. We present the above discussion as a hypothesized mechanism for sensitized TiO 2 solar cell degradation in the absence of oxygen and acknowledge that further studies are required to definitively establish the mechanism. Interestingly, acetonitrile has been shown to pacify Ti 3+ oxygen vacancy sites in TiO 2 (refs 32 , 33 ). This may explain why this rapid UV degradation has not been reported for liquid electrolyte DSSCs using nitrile-based solvents, although as mentioned earlier, UV cutoff filters are usually used during long-term stability measurements [44] , [45] , [46] , [47] , [48] . 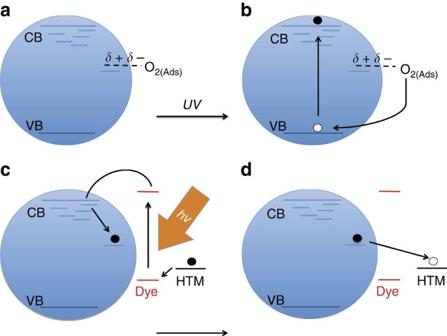Figure 5: Proposed mechanism for UV-induced degradation. Upon UV light exposure, the photogenerated holes react with the oxygen radicals adsorbed at surface oxygen vacancies (a,b). Molecular oxygen is desorbed from these sites, leaving unoccupied, deep surface traps sites and a free electron per site. These electrons will recombine with the excess of holes in the doped-hole transporter. Upon photo excitation of the sensitizer, electrons are injected either (1) into the conduction band from which they become deeply trapped or (2) directly into the deep surface traps (c). These deeply trapped electrons are not mobile and recombine readily with holes on the spiro-OMeTAD hole transporter (d). Figure 5: Proposed mechanism for UV-induced degradation. Upon UV light exposure, the photogenerated holes react with the oxygen radicals adsorbed at surface oxygen vacancies ( a , b ). Molecular oxygen is desorbed from these sites, leaving unoccupied, deep surface traps sites and a free electron per site. These electrons will recombine with the excess of holes in the doped-hole transporter. Upon photo excitation of the sensitizer, electrons are injected either (1) into the conduction band from which they become deeply trapped or (2) directly into the deep surface traps ( c ). These deeply trapped electrons are not mobile and recombine readily with holes on the spiro-OMeTAD hole transporter ( d ). Full size image Having established that TiO 2 -based solar cells have an inherent instability under UV illumination, there are several options to overcome this: either develop a route to effectively and stably pacify the TiO 2 surface states in the solid state, or prevent the UV light from reaching the mesoporous TiO 2 while still using it to generate photocurrent, or completely remove the mesoporous TiO 2 . With regard to the second option, down-converting nanoparticles have been demonstrated to efficiently absorb UV light and re-emit visible light that can be harvested by the sensitizer in DSSCs [49] , [50] . Developing such routes to harvest all of the light of shorter wavelengths than 435 nm before it reaches the mesoporous TiO 2 , should allow for enhanced stability without the cost of decreased photocurrents [49] , [50] . With regard to removing the TiO 2 altogether, we have recently developed perovskite-based MSSCs, within which the mesoporous n-type TiO 2 is replaced with an insulating mesoporous Al 2 O 3 scaffold ( Fig. 1b ) [8] , [11] . In Fig. 6 we show the device performance parameters, measured every 15 min whilst exposing the MSSCs to continuous simulated AM 1.5 76.5 mW cm −2 illumination at 40 °C with no UV cutoff filter present. It is quite evident that the perovskite MSSCs are indeed considerably more resilient to UV irradiation than the perovskite-sensitized TiO 2 analogue. Contrary to the behaviour observed for TiO 2 -based cells under UV light exposure (almost complete decay within 3 h), the photocurrent remains stable at close to 15 mA cm −2 over the 1,000 h exposure period. There is some initial deterioration in the fill factor and open-circuit voltages of the cells over the first 200 h of exposure. This could be due to a number of factors including: partial de-doping of the spiro-OMeTAD hole conductor [15] , oxygen desorption at vacancy sites on the remaining TiO 2 compact layer, changes to the spiro-OMeTAD–Au electrode contact, or indeed some subtle changes within the perovskite absorber. However, we have previously demonstrated the optical stability of the mixed halide perovskite under full spectrum simulated sunlight and see no change to the optical absorption spectrum [8] , so it does not appear that this contributes to the initial degradation. This is supported by the lack of degradation in photocurrent over the first several 100 h. The rudimentary encapsulation technique we have employed, using epoxy resin may also induce some degradation due to migration of reactants into the photoactive layer. The possible sources of and mechanism for the longer-term changes are currently under intensive investigation. Our results however show that following the initial drop within the first 200 h, a stable power conversion efficiency of approximately 6% is achieved which subsequently remains constant throughout the 1,000 h. This is already superior to any results obtained either in our laboratory or from the literature when using TiO 2 as the electron transporter in solid-state SSCs [15] , [16] , [17] . We note that a recent study by Burschka et al. demonstrated methylammonium lead tri-iodide sensitized TiO 2 solar cells to be stable up to 500 h [9] , but this was accomplished under white light emitting diodes in the absence of UV light, so we expect such cells to suffer from the same UV sensitivity as we observe here for our sensitized TiO 2 solar cells. 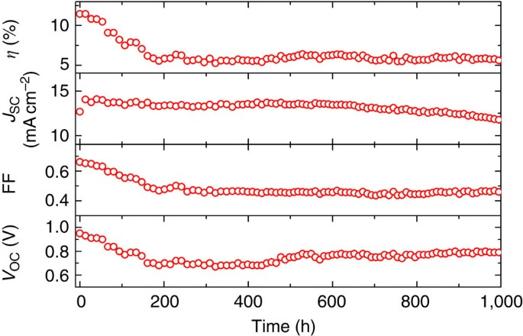Figure 6: 1,000 h stability plot of MSSC mesoporous TiO2-free solar cells. Solar cell performance parameters measured directly during aging of a representative Al2O3-based perovskite solar cell monitored every 15 min under continuous illumination of approximately one sun light intensity (actual intensity 76.5 mW cm−2) at 40 °C (Atlas CPSPlus Xenon lamp aging box). The device was encapsulated with epoxy resin and a glass coverslip in a nitrogen-filled glove box and no UV cutoff filters are used. Figure 6: 1,000 h stability plot of MSSC mesoporous TiO 2 -free solar cells. Solar cell performance parameters measured directly during aging of a representative Al 2 O 3 -based perovskite solar cell monitored every 15 min under continuous illumination of approximately one sun light intensity (actual intensity 76.5 mW cm −2 ) at 40 °C (Atlas CPSPlus Xenon lamp aging box). The device was encapsulated with epoxy resin and a glass coverslip in a nitrogen-filled glove box and no UV cutoff filters are used. Full size image We moreover point out that while the sensitized TiO 2 -based solar cells appear to be more stable when a UV filter is used, this comes at a cost of photocurrent, and requires an extremely stable and cheap UV filter. In addition, since the absorption tail of mesoporous TiO 2 extends into the visible, there may be degradation over a longer timescale due to absorption in the tail [51] . We do indeed observe that the encapsulated TiO 2 -sensitized cells tested beneath a 435-nm cutoff filter do degrade to approximately 85% of their initial performance over the first 4 h ( Fig. 2 ), whereas the TiO 2 -free solar cells are perfectly stable (and even improve) over this short time period ( Fig. 6 ). We have then been able to identify a major instability of solid-state sensitized TiO 2 -based solar cells; they are unstable to UV illumination when encapsulated in an inert atmosphere. Unless addressed, such instability will inhibit commercial deployment of these solar cells. The Al 2 O 3 -based MSSCs circumvent this inherent instability, and display stable photocurrents under continuous full spectrum sunlight for a period of over 1,000 h. Though this is only the first step in the path towards the requisite 25-year outdoor operational lifetime, it illustrates that the thin film and meso-superstructured perovskite solar cells have bypassed a critical instability of the mesoporous TiO 2 -based solar cells, and show significant promise as a large scale, long-term energy source. Device fabrication CH 3 NH 3 PbI 3−x Cl x solar cells: The synthesis of the perovskite, CH 3 NH 3 PbI 3− x Cl x , has been reported elsewhere, as has the preparation for the TiO 2 -based solar cells [8] , [11] . Briefly, for the MSSCs, fluorine-doped tin oxide coated glass substrates were cleaned sequentially in Hellmanex, acetone, isopropanol and oxygen plasma. A 50-nm compact layer of TiO 2 was deposited by spin coating (2,000 r.p.m., 2,000 r.p.m. s −1 ramp) a weakly acidic solution of titanium isopropoxide in ethanol (containing 35 μl of 2 M HCL per 5 ml of solution), and sintered at 500 °C for 30 min. The low-temperature Al 2 O 3 scaffold was deposited by spin-coating (speed=2,500 r.p.m., ramp=2,500 r.p.m. s −1 , time=60 s) a colloidal dispersion of<50 nm Al 2 O 3 nanoparticles (Sigma-Aldrich, product number 702129) in isopropanol (1:2 by volume), followed by drying at 150 °C for 10 min, giving a 400-nm scaffold. The perovskite was deposited by spin coating (speed=2,000 r.p.m., ramp=2,000 r.p.m. s −1 , time=60 s) an ~40 wt% DMF solution of methylammonium iodide and PbCl 2 (3:1 molar ratio). The substrate is then heated to 100 °C for 45 min in an oven. The hole-transport layer was deposited by spin coating an 8.5 vol.% 2,2′,7,7′-tetrakis-( N , N -di- p - methoxyphenylamine)9,9′-spirobifluorene (spiro-OMeTAD) in chlorobenzene solution with the standard additives tert-butylpyridine (0.80 mM) and lithium bis(trifluoromethanesulfonyl)imide (20 mM). Gold electrodes were then deposited by evaporation under high vacuum through a shadow mask. For the TiO 2 perovskite-SSCs, the substrate was cleaned and the compact layer deposited as described for the MSSCs. Then 500 nm of mesoporous TiO 2 was deposited by spin coating a solution of dyesol paste (18 NR-T) in a 1:2.5 mass ratio to ethanol at 2,000 r.p.m. with a 2,000 r.p.m. s −1 ramp. This layer was sintered at 550 °C for 45 min. Upon cooling, a 20 wt% solution of the perovskite precursor (described above) was spin coated at 2,000 r.p.m., 2,000 r.p.m. s −1 ramp, to sensitize the TiO 2 . For the devices where the perovskite completely fills the pores, a 1:6 ratio of dyesol paste to ethanol was used, and a 30 wt% solution of perovskite precursors was used. Gold electrodes were deposited on the cells by evaporation. For the simultaneous current extraction and TAS measurements, the gold electrodes were only 15 nm thick, allowing them to be semitransparent. DSSCs were prepared as described elsewhere, using D102 and C106 as the dye sensitizers [25] . Conductivity devices: Conductivity measurements were conducted on devices prepared in the same manner as the dye-SSCs, except that the films are prepared on glass substrates, and that an interdigitated two-point contact mask was used to evaporate the gold contacts, as described elsewhere [27] . In the case where the TiO 2 conductivity was measured, the contacts were evaporated onto the glass, upon which the device was then built, and no hole transporter was deposited on the dye-sensitized film. For measuring the hole transporter conductivity, the photoactive layer of a complete solar cell was prepared on glass, with the appropriate electrodes deposited on the spiro-OMeTAD capping layer [27] . Encapsulation: Devices were prepared in air and then brought into a nitrogen-filled glovebox. They were allowed to rest in the glovebox for 24 h, after which a quick drying two-part epoxy was dropped over the electrodes, and a small glass coverslip placed on top, to seal the devices. Device characterization Current-voltage characteristics were measured under AM 1.5 100 mW cm −2 simulated sunlight (ABET Technologies Sun 2000) with a Keithley 2400. The apparatus for device characterization was calibrated with an NREL certified KG5 filtered Si reference diode. The cell area under test was defined with a square aperture in a metal mask to be 0.09 cm 2 . The short-term stability measurements depicted in Fig. 2 were performed in the same way, where the solar cells were held at open circuit and scanned every 5 min. Aging: The long-term aging measurements were carried out under 100 mW cm −2 light intensity (Atlas CPSPlus Xenon lamp) at 40 °C, where the devices were held at open circuit and tested every 15 min. The simultaneous conductivity measurements and TAS, as well as the simultaneous current extraction and TAS measurements have been reported elsewhere [27] . Here, we used an Nd:YAG laser at 550 nm pump wavelength and laser intensity 35 mJ, which was reduced to around 80 μJ cm −2 using neutral density filters for the current extraction measurements, at 10 ns pulse length and 10 Hz repetition rate, which yielded charge densities similar to those found in the devices under normal operating conditions. How to cite this article: Leijtens, T. et al. Overcoming ultraviolet light instability of sensitized TiO 2 with meso-superstructured organometal tri-halide perovskite solar cells. Nat. Commun. 4:2885 doi: 10.1038/ncomms3885 (2013).